Structural reducibility of multilayer networks Many complex systems can be represented as networks consisting of distinct types of interactions, which can be categorized as links belonging to different layers. For example, a good description of the full protein–protein interactome requires, for some organisms, up to seven distinct network layers, accounting for different genetic and physical interactions, each containing thousands of protein–protein relationships. A fundamental open question is then how many layers are indeed necessary to accurately represent the structure of a multilayered complex system. Here we introduce a method based on quantum theory to reduce the number of layers to a minimum while maximizing the distinguishability between the multilayer network and the corresponding aggregated graph. We validate our approach on synthetic benchmarks and we show that the number of informative layers in some real multilayer networks of protein–genetic interactions, social, economical and transportation systems can be reduced by up to 75%. Network science has shown that characterizing the stucture of a complex system is fundamental when it comes to understanding its dynamical properties [1] , [2] , [3] . In particular, the basic units of most real-world systems are subject to different types of interactions occurring at comparable time scales. For instance, this is the case of social systems, where individuals can have political or financial relationships [4] , or can be interacting using different communication channels, including face-to-face interactions, e-mail, Twitter, Facebook, phone calls and so on [5] , [6] . Similarly, in biological systems basic constituents such as proteins can have physical, co-localization, genetic or many other types of interactions. Recently, it has been shown that retaining such multi-dimensional information [7] and modelling the structure of interdependent and multilayer systems respectively through interdependent [8] and multilayer networks [9] , [10] , [11] , [12] reveals new non-trivial structural properties [13] , [14] , [15] , [16] , [17] , [18] , [19] , [20] and relevant emergent physical phenomena [21] , [22] , [23] , [24] , [25] , [26] , [27] . However, some of the interaction layers considered in the multidimensional representation of a system can be redundant or uninformative. Then, a simple question arises about the possibility of reducing the structure of a multilayer network, that is, of considering a smaller number of layers, while retaining as much information as possible about the whole system. This problem has both theoretical and practical implications. From a theoretical point of view, it is always desirable to find the most economical description of a phenomenon, that is, the one which retains all the salient aspects of the system avoiding unnecessary redundancy. From a practical point of view, the computation of even basic structural descriptors for interdependent and multilayer networks, such as clustering coefficient, centrality, motifs abundance and all the measures based on paths and walks, scales superlinearly or even exponentially with the number of layers [17] and can thus result unfeasible already for medium-sized networks. Therefore, finding an optimal configuration consisting of a minimal number of layers becomes a fundamental requirement when dealing with real-world systems. Inspired by a similar question arising in quantum physics when one needs to quantify the distance between mixed quantum states [28] , we propose here a method to aggregate some of the layers of a multilayer system while maximizing its distinguishability from the aggregated network. The method is based on a purely information theoretic perspective, which makes use of the definition of Von Neumann entropy of a graph. We test our procedure on synthetic and real-world multilayer networks, showing that different levels of structural reduction are possible, depending on the overall organization of the network. Von Neumann entropy of a multilayer network In quantum mechanics, there are pure states, describing the system by means of a single vector in the Hilbert space, and mixed states, corresponding to statistical ensembles of pure states. The most general quantum system can then be described by the so-called density operator ρ , a semidefinite positive matrix with eigenvalues summing up to 1, which encodes all the information about the statistical ensemble of pure states of the system [29] . The Von Neumann (entanglement) entropy, which is the natural extension of the Shannon information entropy to quantum operators, is a widely adopted descriptor to measure the mixedness of a quantum system, although other measures, satisfying extensivity or non-extensivity, have been lately introduced and studied [30] . The Von Neumann entropy is defined for any density operator ρ . In particular, if the Von Neumann entropy is zero the system is in a pure state, otherwise it is in a mixed state. In general, the larger the Von Neumann entropy, the more mixed the state is. It has been recently shown that the Von Neumann entropy can also be used to characterize (single layer) graphs [31] , [32] . Given a graph G represented by the adjacency matrix A , the Von Neumann entropy of G is defined as the Shannon entropy of the spectrum of the rescaled combinatorial Laplacian associated to G (see Methods). This entropy has been interpreted as the entanglement of the statistical ensemble of pure states where each pure state is one of the edges of the graph [33] . According to this interpretation, a graph is in a pure state if and only if it consists of exactly one edge, corresponding to a Von Neumann entropy h A =0, and is in a mixed state otherwise, yielding h A >0. Here we use a similar formalism to characterize multilayer networks, where we assume that each layer represents one possible state of the system, that is, a network state. We propose to use the Von Neumann entropy to quantify the distinguishability between a multilayer network (or a reduced configuration of its original layers) and the network obtained by aggregating all its layers in a single-layer graph. Let us consider a multilayer network with the N nodes replicated along the different layers [12] . Such a network can be represented by the set , whose elements are the N × N adjacency matrices of the M layers [11] , [17] . This particular multilayer structure is known as multiplex in the literature [12] . We define the Von Neumann entropy of a multilayer network as the sum of the Von Neumann entropies of its M layers, that is, where and are the eigenvalues of the rescaled Laplacian matrix associated to the adjacency matrix A [ α ] of layer α (see Methods). In the case of more general multilayer networks, where more complicated patterns of interlayer connections are allowed, it is still possible to calculate the Von Neumann entropy by considering the supra-adjacency matrix introduced by Gomez et al . [21] , obtained as a special flattening of the rank-4 adjacency tensor, an even more general representation of multilayer networks [10] . Quantifying the reducibility of a multilayer network The Von Neumann entropy of a multilayer network explicitly depends on the actual number of layers M and on the structure of each layer, so that in general its value will change if we consider a reduced multilayer network in which some of the layers of the original system have been combined together by means of an appropriate aggregation method. A particular case is represented by the aggregated graph associated to , which is the one-layer network whose adjacency matrix A is obtained by summing the adjacency matrices of all the M layers of , that is, A = A [1] + A [2] +…+ A [M] . The Von Neumann entropy of the aggregated graph is h A . In general, if we start from an M layer multiplex network and aggregate some of the original layers of , we obtain a reduced multilayer network with X ≤ M layers, where the adjacency matrix C [ α ] , where α =1,…, X is either one of the adjacency matrices of the original layers of or the sum of two or more of them. We then consider the entropy per layer of the multilayer network : and we propose to quantify the distinguishability between the multilayer network and the corresponding aggregated graph A through the relative entropy: The larger , the more distinguishable is the multilayer network from the corresponding aggregated graph A . It is worth noting that if all the layers of the multilayer network are identical, then , as and the aggregated graph are totally equivalent. Conversely, a value indicates that the representation with X layers is distinguishable from the aggregated one; hence the multilayer structure must be preserved. Intuitively, if the aggregation of two layers does not result in a decrease of the relative entropy with respect to the multiplex in which the two layers are kept separated, then one would prefer the reduced configuration, which is more compact. However, it is possible to show (see Methods) that if we consider a multilayer with X layers and the reduced configuration with X –1 layers obtained from by aggregating two of its layers, then in general can be smaller than, equal to, or even larger than . This is due to the fact that the entropy per layer can either increase or decrease as a consequence of the aggregation of two layers (see Supplementary Fig. 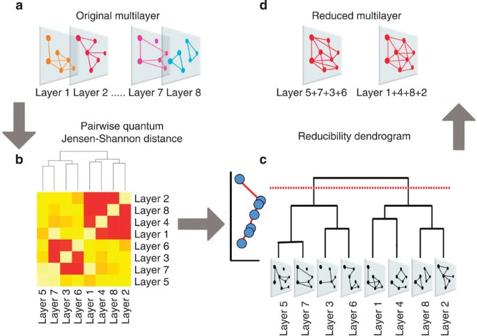Figure 1: Layer aggregation and structural reducibility of multilayer networks. Given a multilayer network (a), we compute the Jensen–Shannon distancebetween each pair of its layers (b), which is a proxy for layer redundancy. Such resulting distance matrix allows to perform a hierarchical clustering, whose output is a hierarchical diagram (a dendrogram) whose leaves represent the initial layers and internal nodes denote layer merging (c). At each step, the two clustered layers (or group of layers) corresponding to the smallest value ofare aggregated and the quality of the new layer configuration in terms of distinguishability from the aggregated graph is quantified by the global quality functionq(·), shown by the curve on the left-hand side ofc. The best partition is the one for whichq(·) is maximal (d). 1 and Supplementary Table 1 ). As we show in detail in Methods, our goal is to find argmax , that is, the optimally reduced multiplex yielding the maximum value of distinguishability from the aggregated graph. If we denote by M opt the number of layers corresponding to the maximum value of relative entropy max[ q (·)], we can then define the reducibility of a multilayer network as: which is the ratio between the number of reductions ( M – M opt ) and the total possible number of potentially reducible layers ( M –1). It is worth noting that if the system cannot be reduced, that is, when M opt = M , while only if M opt =1, that is, if the M layers can indeed be reduced into a single one (that is, the aggregated network). The optimal configuration of aggregated layers is the one that maximizes the relative entropy q (·), but finding such a configuration would in general require the enumeration of all the possible partitions of a set of M objects (the layers), which is a well-known NP-hard problem (that is, its solution requires a computational time that scales at least exponentially with M ). To overcome this problem, we adopt a greedy agglomerative hierarchical clustering algorithm [34] to explore the space of partitions, based on a concept of distance similar to the one adopted in quantum physics to quantify the distance between mixed quantum states [28] . More specifically, capitalizing on the concept of Von Neumann entropy of a graph, we use the quantum Jensen–Shannon divergence to quantify the (dis-)similarity between all pairs of layers of a multilayer network (see Methods). At each step of the algorithm, we consider the pair of layers having the smallest value of quantum Jensen–Shannon divergence and we aggregate them, obtaining a new multilayer network with one layer less. The rationale behind this choice is that the aggregation of a pair of similar layers is more desirable than the aggregation of two very dissimilar layers, as the latter can introduce artificial structural patterns. The result of this procedure is a dendrogram (see Fig. 1 ), that is, a hierarchical diagram where each of the M leaves is associated to one of the original layers of the system, each internal node indicates the aggregation of layers (or of clusters of layers) together and the root corresponds to the fully aggregated graph. At the m th step of the algorithm, we obtain a multilayer with M – m layers, for which we can compute the associated value of relative entropy q (·). The cut of the dendrogram corresponding to the maximal value of q (·) identifies the (sub-)optimal configuration of layers in terms of distinguishability with respect to the aggregated graph. The whole procedure proposed is sketched in Fig. 1 and can be summarized as follows: (i) compute the quantum Jensen–Shannon distance matrix between all pairs of layers; (ii) perform hierarchical clustering of layers using such distance matrix and use the relative entropy q (·) as the quality function for the resulting partition; (iii) finally, choose the partition that maximizes the relative entropy, that is, the distinguishability from the aggregated graph. Figure 1: Layer aggregation and structural reducibility of multilayer networks. Given a multilayer network ( a ), we compute the Jensen–Shannon distance between each pair of its layers ( b ), which is a proxy for layer redundancy. Such resulting distance matrix allows to perform a hierarchical clustering, whose output is a hierarchical diagram (a dendrogram) whose leaves represent the initial layers and internal nodes denote layer merging ( c ). At each step, the two clustered layers (or group of layers) corresponding to the smallest value of are aggregated and the quality of the new layer configuration in terms of distinguishability from the aggregated graph is quantified by the global quality function q (·), shown by the curve on the left-hand side of c . The best partition is the one for which q (·) is maximal ( d ). Full size image Reduction of synthetic multilayer networks To shed light on the impact of the structural properties of a multilayer network on the results obtained through the proposed layer reduction procedure, we considered different synthetic multilayer benchmarks. Each benchmark consists of several layers characterized by specific features or by a given amount of correlation. In Fig. 2 we report the case of a multilayer network in which the layers are obtained by rewiring different percentages of the edges of the same original layer. The layers of the resulting multilayer network are characterized by an increasing amount of edge overlap (see Methods). As shown in the figure, the hierarchical clustering procedure first aggregates layers characterized by smaller rewiring, which are more similar to each other, and then proceeds to the aggregation of layers obtained for larger values of rewiring. The monotonically decreasing behaviour of the relative entropy q (·), shown in Fig. 2c , confirms that in this case the best representation of the system is the one in which all the layers are kept distinct. In fact, independently of the fraction of edges actually rewired, on average a pair of layers exhibits a relatively small redundancy, as each of the rewired layers carries some information that is not included in the other layers (this multilayer has an overall edge overlap smaller than 5%). 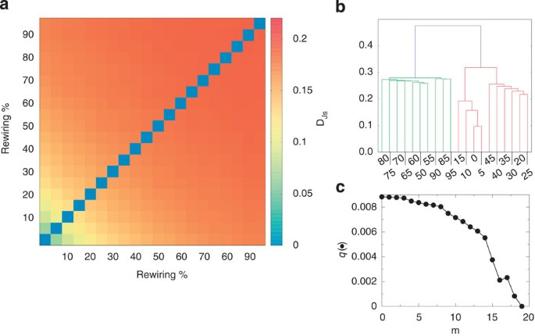Figure 2: Multilayer benchmark. We considered a benchmark multilayer network withN=5,000 nodes andM=20 layers. The first layer is a scale-free graph withP(k)∼k−3, whereas the other layers are obtained by rewiring an increasing percentage of the edges of the first layer, from 5% up to 95%. By doing so, each pair of layers is characterized by a different amount of edge redundancy (the total overlap of the multilayer is <5%). (a) The heat map shows the Jensen–Shannon distance between the 20 layers, where each layer is identified by the corresponding percentage of rewiring. (b) The hierarchical clustering procedure successively merges layers with a decreasing percentage of redundant edges. (c) In this caseq(·) is a decreasing function ofm, as each layer has some unique edges that are not present in the others. The best representation of the multilayer is that in which all the layers are kept separated, even ifq(·) remains almost constant in the first few aggregation steps (corresponding to the aggregation of pairs of layers with a rewiring smaller than 15%). Figure 2: Multilayer benchmark. We considered a benchmark multilayer network with N =5,000 nodes and M =20 layers. The first layer is a scale-free graph with P ( k ) ∼ k −3 , whereas the other layers are obtained by rewiring an increasing percentage of the edges of the first layer, from 5% up to 95%. By doing so, each pair of layers is characterized by a different amount of edge redundancy (the total overlap of the multilayer is <5%). ( a ) The heat map shows the Jensen–Shannon distance between the 20 layers, where each layer is identified by the corresponding percentage of rewiring. ( b ) The hierarchical clustering procedure successively merges layers with a decreasing percentage of redundant edges. ( c ) In this case q (·) is a decreasing function of m , as each layer has some unique edges that are not present in the others. The best representation of the multilayer is that in which all the layers are kept separated, even if q (·) remains almost constant in the first few aggregation steps (corresponding to the aggregation of pairs of layers with a rewiring smaller than 15%). Full size image The results obtained on several other synthetic multilayer networks suggest that layers with high edge overlap and similar structure, for example, characterized by highly overlapping communities, tend to be aggregated earlier (see Supplementary Note 1 , Supplementary Figs 2,3 and 4 ). Reduction of multilayer biological networks To test the usefulness of our method on real-world systems, we consider here the multilayer networks obtained by taking into account different types of genetic interactions in 13 organisms of the Biological General Repository for Interaction Datasets (BioGRID [35] ). This is a public database that stores and disseminates genetic and protein interaction information about simple organisms and humans ( http://thebiogrid.org ), and currently holds over 720,000 interactions obtained from both high-throughput data sets and individual focused studies, as derived from over 41,000 publications in the primary literature. We use BioGRID 3.2.108 (updated to 1 Jan 2014). In this data set, the networks represent protein–protein interactions and the layers correspond to interactions of different nature, that is, physical (labelled ‘Phys’ in the following), direct (‘Dir’), co-localization (‘Col’), association (‘Ass’) and suppressive (‘GSup’), additive (‘GAdd’) or synthetic genetic (‘GSyn’) interaction. The number of layers identified for each organism ranges from three to seven. In Fig. 3 we show the results obtained on three organisms ( Caenorhabditis elegans , Mus and Candida ). Despite the multilayer networks corresponding to these organisms have a similar number of layers (six for C. elegans , seven for Mus and Candida ), each of them is characterized by a peculiar level of structural reducibility. In particular, in the case of C. elegans no layer aggregation is possible at all, as the maximum value of q (·) is obtained for the multilayer in which all the six layers are kept distinct. Hence, the reducibility is . Conversely, in the case of Mus and Candida some pairs of layers carry redundant structural information and can be thus aggregated. Remarkably, the reducibility for Candida is , corresponding to three redundant interaction layers out of seven. Here, the layer associated to genetic synthetic interactions is first aggregated with the layer encoding genetic additive interactions, while direct interactions are aggregated with physical ones. For other organisms, the value of reducibility can be as high as (see Table 1 for details). 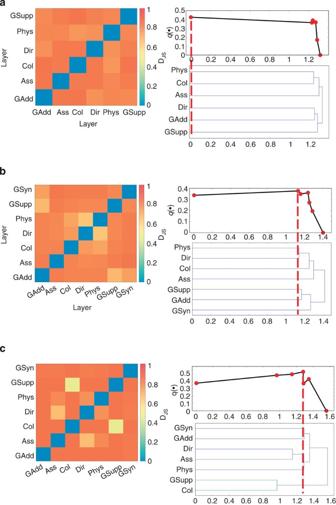Figure 3: Layer aggregation of protein–genetic interaction networks. The multilayer protein–genetic networks of different species have different levels of reducibility. We show the heat map of the Jensen–Shannon divergence, together with the dendrogram resulting from hierarchical clustering and the corresponding values ofq(·), in 3 of the 13 species considered in this study. The dashed red lines identify the maximum of the global quality functionq(·). For some organisms (such asC. elegans, reported ina), such maximum is obtained by leaving all the layers separate and no aggregation is possible, whereas for some other species a few layers carry redundant information, for example, in (b)Musand in (c)Candida. Figure 3: Layer aggregation of protein–genetic interaction networks. The multilayer protein–genetic networks of different species have different levels of reducibility. We show the heat map of the Jensen–Shannon divergence, together with the dendrogram resulting from hierarchical clustering and the corresponding values of q (·), in 3 of the 13 species considered in this study. The dashed red lines identify the maximum of the global quality function q (·). For some organisms (such as C. elegans , reported in a ), such maximum is obtained by leaving all the layers separate and no aggregation is possible, whereas for some other species a few layers carry redundant information, for example, in ( b ) Mus and in ( c ) Candida . Full size image Table 1 Reducibility of empirical multilayer networks. Full size table In Fig. 4 we summarize the results obtained by applying the proposed layer aggregation procedure to all the 13 multilayer genetic interaction networks of the BioGRID data set. This particular visualization allows to compare the structural reducibility of all organisms simultaneously. Not all multilayer networks can be reduced to a smaller number of layers, suggesting that for some organisms layer aggregation should be avoided. For instance, this is the case of C. elegans (nematode), Arabidopsis thaliana (cress) and Bos taurus (mammal), where no global maximum is present, except for m =0, that is, the initial multilayer in which all layers are kept distinct. In other cases, some of the layers are clearly redundant, as happens for instance in Saccharomyces cerevisiae (yeast) and Drosophila melanogaster (common fruit fly), where a maximum of q (·) is present at m =2. 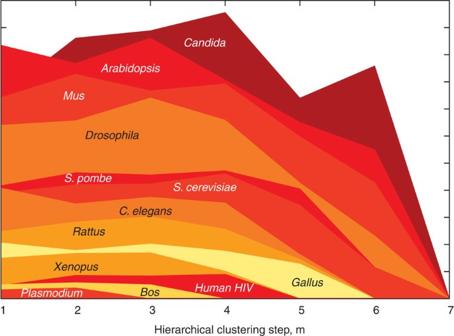Figure 4: Structural reducibility of protein–genetic networks in the BioGRID data set. The global quality functionq(·) versus the number of merges in the hierarchical clustering procedure for the protein–genetic interaction multilayer networks of all the 13 organisms considered in this study (the plots are vertically rescaled to avoid overlaps). The values ofq(·) are not reported in theyaxis, because only the existence of a global maximum, and the corresponding value ofmin thexaxis is meaningful for the analysis. For each organism,q(·) has a maximum corresponding to the partition of the layers which minimizes layer redundancy at the cost of a small loss of information. Figure 4: Structural reducibility of protein–genetic networks in the BioGRID data set. The global quality function q (·) versus the number of merges in the hierarchical clustering procedure for the protein–genetic interaction multilayer networks of all the 13 organisms considered in this study (the plots are vertically rescaled to avoid overlaps). The values of q (·) are not reported in the y axis, because only the existence of a global maximum, and the corresponding value of m in the x axis is meaningful for the analysis. For each organism, q (·) has a maximum corresponding to the partition of the layers which minimizes layer redundancy at the cost of a small loss of information. Full size image Note that the reducibility values obtained for the above mentioned biological networks are conditioned to the completeness of the corresponding data sets. As a matter of fact, although the protein interactions of some organisms are well known and thoroughly characterized as in the case of S. cerevisiae or D. melanogaster , for some other organisms the information is only partial or incomplete. Hence, we cannot estimate a priori how the partial information contained in these networks is indeed affecting the values of reducibility that we observe. Nowadays, larger and more detailed data sets describing diverse natural and man-made systems are being produced at an increasingly fast rate. This data deluge has provided an unprecedented amount of information about social, biological and technological phenomena, allowing a better characterization of the structure of different complex systems and a more in-depth understanding of the mechanisms underpinning their functioning. On the one hand, multilayer networks represent a natural framework to properly take into account all the different kinds of relationships connecting the units of a system, in a coherent manner. On the other hand, dealing with multilayer graphs introduces new computational challenges, which might limit the applicability of the multilayer approach to large systems. As a matter of fact, the evaluation of the multilayer version of even the most basic network descriptors, such as average shortest path length, node clustering coefficient, node betweenness and network motifs, tend to scale exponentially with the number of layers of the system and might become too computationally demanding already for medium-sized systems. A fundamental observation is that not all the available levels of interaction among the constituents of a complex system have the same importance and some of them might be redundant, irrelevant or uninformative, with respect to the overall structure of the system. Hence, comes the idea of providing a consistent way to aggregate some of the layers of a multilayer network according to their similarity, as measured by the quantum Jensen–Shannon divergence, and of looking for configurations of layers that guarantee the maximum possible distinguishability from the fully aggregated graph and still use a minimal number of layers. The proposed approach allows to effectively reduce the redundancy of a multilayer network, as extensively shown in the paper for the case of the protein–genetic interaction networks of several different species. However, the applicability of this method is not limited to biological systems. As an example, we have applied it also to social [17] and economical systems, coauthorship networks [36] , metropolitan transportation networks [24] and continental air transportation systems [20] (see Table 1 ). A particularly interesting case is that of the FAO (Food and Agriculture Organization of the United Nations) worldwide food import/export network, an economic network in which layers represent products, nodes are countries and edges at each layer represent import/export relationships of a specific food product among countries. We collected the data from http://www.fao.org and built the multilayer network corresponding to trading in 2010. In Fig. 5 we show the distance matrix and the network visualization of three representative layers. The hierarchical clustering procedure reveals that up to 158 out of the 340 available layers can indeed be reduced, yielding a value of close to 50%. Intriguingly, the layers that are aggregated in the earlier stages of the clustering procedure correspond to products characterized by similar import/export patterns, as happens for instance for the layers associated to nuts, cocoa, dried and prepared fruits, roasted coffee and coffee-related products, which mainly involve export from Australia, China and Africa to European countries and the United States. 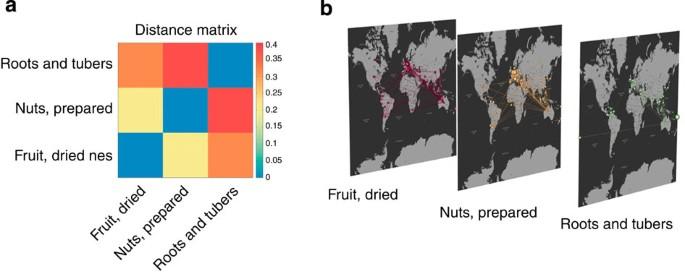Figure 5: Structural reducibility of the FAO worldwide food import/export network. The distance matrix of three layers of the FAO worldwide food import/export data set, corresponding to three specific products (that is, ‘roots and tubers’, ‘prepared nuts’ and ‘dried fruit’), is shown ina, whereas the topology of the three layers is reported inb. The layers corresponding to ‘prepared nuts’ and ‘dried fruits’, which are more similar to each other (that is, closer with respect to the Jensen–Shannon divergence), are indeed aggregated by the algorithm in a single cluster, whereas the ‘roots and tubers’ layer, which is characterized by a remarkably different topology as evident fromb, is kept separated. Map tiles By Stamen Design, under CC BY 3.0. Data by OpenStreetMap, under CC BY SA. Figure 5: Structural reducibility of the FAO worldwide food import/export network. The distance matrix of three layers of the FAO worldwide food import/export data set, corresponding to three specific products (that is, ‘roots and tubers’, ‘prepared nuts’ and ‘dried fruit’), is shown in a , whereas the topology of the three layers is reported in b . The layers corresponding to ‘prepared nuts’ and ‘dried fruits’, which are more similar to each other (that is, closer with respect to the Jensen–Shannon divergence), are indeed aggregated by the algorithm in a single cluster, whereas the ‘roots and tubers’ layer, which is characterized by a remarkably different topology as evident from b , is kept separated. Map tiles By Stamen Design, under CC BY 3.0. Data by OpenStreetMap, under CC BY SA. Full size image Conversely, the number of layers in the multilayer networks of airline transportation systems cannot be substantially reduced (the few allowed aggregations correspond to layers associated to very small companies, operating on just one or two routes), in agreement with the fact that airline companies tend to minimize the overlap of routes with other operators, to avoid strong competition. This result indicates that the connectivity among airports is practically not redundant for any airline, as expected for a modern large-scale transport infrastructure. Similar results are obtained for the London metropolitan transportation network, in which the overlap among different lines is purposely avoided to guarantee a more efficient coverage of the metropolitan area. In this case, the optimal solution corresponds to the multiplex network in which all the transportation lines are kept separated, with the only exception of the Circle Line and the Hammersmith and City Line, which, as expected, are aggregated together, as they considerably overlap in Zone 1 and Zone 2 (they actually share the same tracks and stations between Hammersmith and Liverpool Street). We would like to clearly point out that by quantifying the reducibility of a multilayer network one obtains information about the structural redundancy of the different layers of the system. However, in the particular case in which the interaction layers are functionally similar, as in the case of unimodal transportation networks or multidisciplinary collaboration networks (but not for gene–protein interaction networks), the optimal multilayer network resulting from the reduction procedure proposed in the study might be also employed, at least to some extent, to characterize the dynamical behaviour of the system. We are confident that this aspect will be the subject of further research in the field. It is worth noticing that although the problem of reducing the number of layers of a multilayer network can be tackled from different perspectives and might in principle be solved using different techniques (most of which are still to be explored), the framework provided by the Von Neumann entropy of graphs allows to formulate this problem in a natural way, and to use a standardised set of tools –borrowed from quantum physics– to define similarity relationships among layers (in terms of Jensen–Shannon divergence) and to construct a quality function able to identify optimal configurations of layers in terms of distinguishability from the aggregated graph. We would also like to stress that the problem of obtaining more compact representations of multilayer networks is interesting per se and we expect that the present work will trigger the investigation of more sophisticated methods for its solution. Beyond the structural reducibility, the reducibility of a multilayer network, while preserving its dynamics and function, remains an outstanding research problem [37] , [38] , [39] . We find quite remarkable that the formal analogy between quantum systems and multilayer networks allows to formulate the problem of layer reducibility in terms of quantum entropy divergence, and we believe that this analogy should be further exploited, as it might effectively provide a novel perspective on the characterization of the structure of multilayer complex systems. Von Neumann entropy of single-layer networks Given a graph G(V, E) with N= | V | nodes and K= | E | edges, represented by the adjacency matrix A= { a ij }, where a ij =1 if node i and node j are connected through an edge, the Von Neumann entropy of G is defined as: where is the combinatorial Laplacian associated to the graph [31] G rescaled by and D is the diagonal matrix of the degrees of the nodes. Formally, has all the properties of a density matrix (that is, it is positive semi-definite and ) and it is easy to prove that h can be written in terms of the set of eigenvalues of : that is, the Von Neumann entropy of a density matrix corresponds to the Shannon entropy of its power spectrum. In Supplementary Methods and Supplementary Fig. 5 we discuss an efficient procedure to approximate the Von Neumann entropy of a graph that avoids the computation of the whole spectrum of . Jensen–Shannon distance between graphs Given two density matrices ρ and σ , it is possible to quantify to which extent ρ is different from σ by means of the Kullback–Liebler divergence: which represents the information gained about σ when the expectation is based only on ρ . However, is not a metric, as it is not symmetric with respect to its arguments (that is, ) and it does not satisfy the triangular inequality. A more suitable quantity to measure the dissimilarity between two density operators is the Jensen–Shannon divergence. If we call the new density matrix obtained as the mixture of the two operators, the Jensen–Shannon divergence between ρ and σ is defined as: By definition, is a reflexive and symmetric relation. In addition, it is possible to prove that , usually called Jensen–Shannon distance, takes values in [0,1] and satisfies all the properties of a metric if applied to qbits [40] . Some recent numerical arguments [41] have shown that behaves similar to a metric as well, when applied to any pair of mixed quantum states, although a rigorous proof is still lacking. We decided to employ the quantum Jensen–Shannon divergence to quantify the distance, in terms of information gain/loss, between the normalized Laplacian matrices associated to two distinct networks. The quality function q (·) The relative entropy defined in equation (2) quantifies the distinguishability of a multilayer network from the corresponding aggregated graph. Here we show that q (·) is an appropriate quality function to maximize, to detect the configuration of layers corresponding to the highest possible distinguishability. In general, q (·) can either increase or decrease as a result of the aggregation of two layers, depending on several factors such as the relative density of the two graphs or their actual wiring patterns. In Supplementary Table 1 we report and discuss several illustrative examples. If we start from the original M -layer multiplex network and aggregate some of its layers, we obtain a new multiplex with X ≤ M layers, where the adjacency matrix of each layer C [ α ] is either one of the adjacency matrices of the original multiplex or the result of the aggregation of two or more of them. In particular, each of the M original layers of will contribute to exactly one of the layers of the reduced multiplex . If we denote by Γ α the layer of the reduced multiplex to which the original layer A [ α ] contributes, then we can express each layer of as where if either the original layer A [ α ] has been aggregated with other layers to form the new layer or if . If we consider the multilayer network with X layers and the reduced multilayer network with X –1 layers obtained from as a consequence of the aggregation of two layers, we want to find the conditions under which or, equivalently, . For the sake of simplicity, and without loss of generality, we assume that the reduced configuration is obtained by aggregating layers C [1] and C [2] into a new layer C [1] + C [2] . After some algebra, the inequality reduces to that is, the quality function q (·) increases as a result of the aggregation, if the entropy of the aggregated layers is smaller than the difference between the sum of the entropies of the layers to be aggregated and the entropy per layer before the aggregation. It is useful to rewrite equation (9) as: where Δ H is the difference of entropy due to the aggregation. This means that q (·) increases if the value of Δ H associated to the two aggregated layers is higher than the entropy per layer of the layer configuration before the aggregation. In general, the Von Neumann entropy is sub-additive, meaning that the entropy of a state obtained as the mixing of two other states is smaller than the sum of the entropies of the two original states, that is, . However, as we extensively show in Supplementary Note 2 , Supplementary Fig. 1 and Supplementary Table 1 , this is not always the case when we aggregate two graphs, so that the Von Neumann entropy of the resulting graph can be either larger or smaller than the sum of the Von Neumann entropies of the two original graphs, that is, the aggregation of two layers can sometimes violate sub-additivity. This happens in at least two cases, that is, when one aggregates layers with very different edge densities or when the aggregation would create structural patterns that did not exist in any of the two original layers, which are both examples of undesirable aggregation (see Supplementary Fig. 1 and Supplementary Table 1 ). In such cases, equation (10) is automatically not satisfied (remember that ) and the quality function q (·) decreases. The condition to have an increase of q (·) expressed by equation (9) can be also written in terms of the Jensen–Shannon divergence of the layers to be aggregated. For the sake of simplicity, let us assume that the two layers C [1] and C [2] aggregated to obtain the new configuration have the same number of links. In this case, the inequality in equation (9) is equivalent to where ρ [1] and ρ [2] are the density matrices corresponding to layers C [1] and C [2] , respectively. The first term on the right-hand side of inequality (11) is the entropy per layer of the multilayer network formed by the two layers that have been aggregated, so that the quality function q (·) increases if the difference between the entropy per layer of this smaller multilayer and the entropy per layer of the full multilayer network is larger than the Jensen–Shannon divergence of the density matrices to be aggregated. In the limiting case in which C [1] and C [2] are identical (that is, ), this leads to an increase of q (·) only if , or equivalently if , that is, if the entropy of each of the two layers is larger than the entropy per layer of the multilayer network before the merge. In conclusion, an increase of q (·) usually corresponds either to the aggregation of two layers that do not violate sub-additivity or to the merge of layers having very similar structure. Hence, by maximizing q (·) one tends to avoid layer configurations that might contain spurious structural patterns or redundant layers. Hierarchical clustering We measure the information lost by merging two layers of a multilayer graph in a single network by comparing the Von Neumann entropy of the compressed multilayer network with the original representation. The main hypothesis is that if the value of the Jensen–Shannon distance between the Laplacian matrices associated to layers α and β is small, then the two layers can be safely merged in a single one without loosing too much information. Conversely, if is large, then the two layers provide different information about the relationships among the nodes of the system. In this case, it would be better to leave the two layers separated, as their aggregation will result in a substantial loss of information. We perform a classical hierarchical clustering of the M layers using the Jensen–Shannon distance to quantify the dissimilarity among (clusters of) layers. At each step of the algorithm, we aggregate the two clusters of layers, which are separated by the smallest value of , and then we update the distances between the newly formed cluster and the remaining ones according to Ward’s linkage. By iterating this procedure M –1 times, we obtain a dendrogram, that is, a hierarchical diagram whose M leaves are associated to the original layers of the system, internal nodes indicate merges of (clusters of) layers and the root corresponds to the aggregated graph. The quality of the layer organization obtained after m steps of the hierarchical clustering algorithm is measured by the relative entropy q (·). To verify whether the proposed greedy clustering procedure is able to find good approximations of the real optimal configuration of layers, we compared the solution corresponding to the optimal cut of the dendrogram with the actual optimal configuration of layers of each of the 13 multilayer networks obtained from the BioGRID data set. For each multilayer network, the optimal configuration of layers was found through exhaustive enumeration of all the possible partitions of the set of layers. The results are reported and discussed in Supplementary Note 3 , Supplementary Table 2 and Supplementary Fig. 6 , and confirm that the greedy clustering algorithm performs a quite efficient exploration of the quality function landscape, yielding (sub-)optimal solutions associated to values of q (·) that are between 76% and 100% of the actual global optimum. This is quite a remarkable result, especially if we consider that the greedy algorithm performs only M –1 steps (that is, less than seven steps for all the BioGRID multilayer networks), while the exhaustive exploration of all the partitions of a set of M elements requires a number of operations equal to the M th Bell number, which increases super-exponentially with M . We notice that the same hierarchical clustering algorithm can be potentially applied with any other measure able to quantify the difference between layers, not just with . The only caveat here is that if the employed measure is not a metric then the classical linkage schemes, including Ward’s linkage, cannot be employed directly, so that at each step it is necessary to recompute the distance between the new layer resulting from the last merge and all the remaining layers. A stand-alone implementation of the algorithm for the reduction of multilayer networks described above is available at https://github.com/KatolaZ/multired . Another implementation of the algorithm is already included in muxViz ( https://github.com/manlius/muxViz ), a software for the multilayer analysis of networks. How to cite this article: De Domenico, M. et al . Structural reducibility of multilayer networks. Nat. Commun. 6:6864 doi: 10.1038/ncomms7864 (2015).